Quantum and classical confinement of resonant states in a trilayer graphene Fabry-Pérot interferometer The advent of few-layer graphene has given rise to a new family of two-dimensional systems with emergent electronic properties governed by relativistic quantum mechanics. The multiple carbon sublattices endow the electronic wavefunctions with pseudospin, a lattice analogue of the relativistic electron spin, whereas the multilayer structure leads to electric-field-effect tunable electronic bands. Here we use these properties to realize giant conductance oscillations in ballistic trilayer graphene Fabry-Pérot interferometers, which result from phase coherent transport through resonant bound states beneath an electrostatic barrier. We confine these states by selectively decoupling them from the leads, resulting in transport via non-resonant states and suppression of the giant oscillations. The confinement is achieved both classically, by manipulating quasiparticle momenta with a magnetic field, and quantum mechanically, by locally varying the pseudospin character of the carrier wavefunctions. Our results illustrate the unique potential of trilayer graphene as a versatile platform for electron optics and pseudospintronics. The development of electronic devices with new functionality or improved performance depends on the ability to manipulate carrier degrees of freedom in low dimensional materials in new ways. To this end, graphenes offer an appealing way forward: low electron–phonon coupling enables micron scale ballistic transport even at elevated temperatures [1] , whereas the ambipolar tunability of the charge carrier density allows the realization of new device concepts based on electron optics [2] . Moreover, the emergent pseudospin, which underlies many of the unique properties of graphitic electronic systems [3] , [4] , can be used as a basis for pseudospintronics [5] , [6] , [7] , the lattice analogue of spintronics [8] . Among the family of few-layer graphenes, ABA (or Bernal)-stacked trilayer graphene (TLG) offers an ideal platform for exploring these effects, as the electronic structure consists of both monolayer and bilayer graphene (MLG and BLG)-like electronic bands [9] , [10] , [11] , [12] , [13] , [14] . Crucially, the layered, two-dimensional arrangement of the carbon planes allows both the charge density and carrier ‘flavour’, MLG- or BLG-like, to be varied through the application of out-of-plane electric fields [11] . By varying the sum and difference of electric displacement fields generated by top and bottom electrostatic gates, the charge carriers in TLG can be tuned continuously between three regimes in which the Fermi level lies in a massless MLG-like hole band, a massive BLG-like ambipolar band or a combination of the two (see Supplementary Fig. S1 ). In this article, we use this tunability to control the TLG band structure and pseudospin properties locally in an electronic Fabry-Pérot interferometer geometry to probe both inter- and intra-species-scattering properties. In the interflavour regime, we observe giant conductance oscillations arising from ballistic, phase coherent transport through BLG-like resonant-bound states beneath the electrostatic barrier. We suppress these giant oscillations by selectively decoupling them from the MLG-like leads, resulting in transport via non-resonant states. The decoupling is achieved both classically, by manipulating quasiparticle momenta with a magnetic field, and quantum mechanically, by locally varying the pseudospin character of the carrier wavefunctions. Compared with previous work on pseudospin effects in quasi-ballistic graphene heterostructures [15] , [16] , which were limited to weak effects due to low sample quality, our devices exhibit a quantitatively and qualitatively different interference regime, both through a dramatic increase in sample quality and by exploiting the wide tunability of the TLG electronic structure. 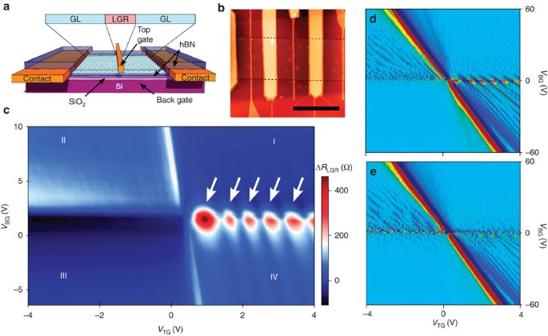Figure 1: TLG heterojunction device schematic and electronic transport measurements. (a) Schematic device representation. A narrow top gate is fabricated on a hBN-encapsulated Bernal-stacked TLG flake. A global, highly doped Si bottom gate controls electron density and the electrical displacement throughout the entire flake, whereas the top gate affects only the LGR. Interfaces between regions of different carrier type can be induced electrostatically at the LGR boundaries by appropriate choice of the top- and bottom-gate voltages. (b) AFM of the measured device. The black dashed lines indicate the TLG edges. Scale bar 4μm. (c) Two terminal resistance data,R, acquired at temperature 300 mK and zero magnetic field. The resistance of the leads has been subtracted by removing a constant resistance corresponding to a uniform channel: ΔRLGR(VBG,VTG)=R(VBG,VTG)−R(VBG,0.37 V), whereVBGis back-gate voltage andVTGis the top-gate voltage. Large amplitude oscillations are visible when the LGR is negatively doped (see arrows). The oscillations decay rapidly for large absolute density in the GLs. (d) Numerical derivative of the two terminal resistance, ∂R/∂VTG, at zero magnetic field. In addition to the giant oscillations, other resonances with smaller amplitude are visible throughout the bipolar regions, II and IV. (e) Numerical derivative of the two terminal resistance at magnetic field 200 mT. Although the small oscillations persist, the giant oscillations are completely suppressed by the classical confinement effect discussed in the main text. Device description Figure 1a shows the device geometry, which consists of an ABA-stacked TLG flake encapsulated by hexagonal boron nitride (hBN). The devices consist of three regions: two outer TLG leads, whose density is controlled by the global bottom gate, and the central locally gated region (LGR), where the density and perpendicular displacement field are independently controlled by the bottom and narrow top gate (see Supplementary Discussion ). The LGR constitutes the electronic Fabry-Pérot cavity. Our hBN-encapsulated samples show low disorder, with mobility μ 60,000 cm 2 V −1 s −1 at 300 mK. The resulting mean free path ( l mf ~600 nm) ensures that the quasiparticles are largely ballistic over length scales comparable to the top-gate width (~60 nm). Figure 1: TLG heterojunction device schematic and electronic transport measurements. ( a ) Schematic device representation. A narrow top gate is fabricated on a hBN-encapsulated Bernal-stacked TLG flake. A global, highly doped Si bottom gate controls electron density and the electrical displacement throughout the entire flake, whereas the top gate affects only the LGR. Interfaces between regions of different carrier type can be induced electrostatically at the LGR boundaries by appropriate choice of the top- and bottom-gate voltages. ( b ) AFM of the measured device. The black dashed lines indicate the TLG edges. Scale bar 4 μ m. ( c ) Two terminal resistance data, R , acquired at temperature 300 mK and zero magnetic field. The resistance of the leads has been subtracted by removing a constant resistance corresponding to a uniform channel: Δ R LGR ( V BG , V TG )=R( V BG ,V TG )−R( V BG ,0.37 V), where V BG is back-gate voltage and V TG is the top-gate voltage. Large amplitude oscillations are visible when the LGR is negatively doped (see arrows). The oscillations decay rapidly for large absolute density in the GLs. ( d ) Numerical derivative of the two terminal resistance, ∂ R /∂ V TG , at zero magnetic field. In addition to the giant oscillations, other resonances with smaller amplitude are visible throughout the bipolar regions, II and IV. ( e ) Numerical derivative of the two terminal resistance at magnetic field 200 mT. Although the small oscillations persist, the giant oscillations are completely suppressed by the classical confinement effect discussed in the main text. Full size image Giant conductance oscillations Fig. 1c shows the change in resistance of the LGR at zero magnetic field as a function of the voltages on the top ( V TG ) and bottom ( V BG ) gates. The contact and graphene lead (GL) resistance, which are independent of V TG , have been substracted from each V BG trace for clarity. The resulting resistance map is divided into four quadrants corresponding to different signs of the charge carrier density in the LGR and GLs [17] , [18] , [19] . The LGR resistance is higher in the bipolar regimes, II and IV, reflecting the presence of electrostatically created pn junctions, and negative in much of regions I and III, reflecting lowered resistance of the LGR when the absolute density is increased locally in the unipolar regime. Figure 1d shows the derivative of the resistance with respect to top-gate voltage, ∂ R /∂ V TG . Small-resistance oscillations arising from phase coherent transport between the pn junctions are visible throughout the bipolar regime. However, unlike electronic Fabry-Pérot resonances in MLG [20] , the TLG data shows an additional set of resistance oscillations with much larger amplitude, visible even in the raw, undifferentiated data (white arrows in Fig. 1c ). In contrast to Fabry-Pérot oscillations in MLG, these oscillations are confined to a narrow region of the V TG − V BG plane and are present only for very low magnetic fields (see Fig. 1e ). These giant oscillations were observed in multiple ABA TLG devices, and are a robust phenomenon, surviving to temperatures as high as ~50 K (see Supplementary Fig. S3 ). Finite element electrostatic simulations of the density and electric displacement field profile along the device, combined with a tight binding analysis of the ABA TLG band structure (see Supplementary Methods ), show that the giant oscillations are observed only when the Fermi level in the GLs lies in the isolated MLG-like hole band, whereas that in the LGR, lies in a BLG-like electron band (see Fig. 2a , inset). This regime, which corresponds to an ‘interflavour’ MLG–BLG heterointerface, is not experimentally realizable in either MLG or BLG. Below, we trace the origin of the giant oscillations to phase coherent transport through a small set of low transverse momentum resonant barrier states (RBS) in the LGR. Remarkably, the presence of the giant oscillations in the conductance is sensitive to the pseudospin character of the charge carriers in the GLs. Their decay with increasing GL density correlates with the population of a BLG-like band in the GLs. In the resulting BLG–BLG interface, normally incident, forward propagating states on opposite sides of the pn junctions are pseudospin mismatched, and the RBS decouple from the GLs states and no longer manifest in transport. In addition to this chirality-assisted confinement of the RBS [21] , the RBS can also be decoupled classically using an external magnetic field, which induces a momentum mismatch between the RBS and the available states in the GLs. We quantitatively describe both decoupling regimes, in which transport is diverted to other diffusive and ballistic channels and the giant oscillations disappear. 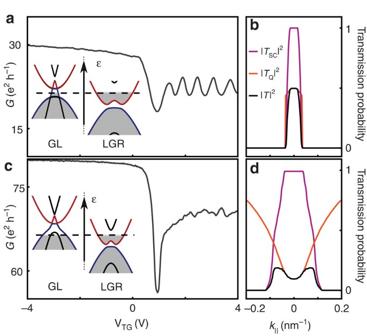Figure 2: Quantum confinement of the RBS. (a) Conductance,G, as function of top-gate voltage (VTG) at back-gate voltage (VBG) −1.6 V, showing large amplitude oscillations. The oscillations are observed when the GLs are populated by MLG-like p-type carriers, whereas the LGR contains BLG-like n-type carriers (inset toa). (b) Calculated transmission probability at a single pn interface in the giant oscillation regime. Interspecies quantum matrix elements do not have a strong parallel momentum (k||) dependence, and the Fermi surface mismatch injects carriers preferentially into the lowk||RBS, leading to the giant oscillations. (c) Conductance as function ofVTGatVBG=−10 V, showing the chirality-assisted decoupling regime. The interface separates BLG-like electron and hole-doped regions (inset), and the measured conductance shows only small-amplitude fluctuations (see alsoSupplementary Fig. S4). (d) Calculated transmission probability at a single pn interface for the electrostatic conditions in (c). In this regime, transmission probability is dominated by BLG–BLG anti-Klein tunnelling: the pseudospin mismatch betweenk||=0 holes in the GL andk||=0 electrons in the LGR suppresses transmission through the RBS28, resulting in a dip in the normal transmission probability and, ultimately, the suppression of the giant oscillations. Figure 2: Quantum confinement of the RBS. ( a ) Conductance, G , as function of top-gate voltage ( V TG ) at back-gate voltage ( V BG ) −1.6 V, showing large amplitude oscillations. The oscillations are observed when the GLs are populated by MLG-like p-type carriers, whereas the LGR contains BLG-like n-type carriers (inset to a ). ( b ) Calculated transmission probability at a single pn interface in the giant oscillation regime. Interspecies quantum matrix elements do not have a strong parallel momentum ( k || ) dependence, and the Fermi surface mismatch injects carriers preferentially into the low k || RBS, leading to the giant oscillations. ( c ) Conductance as function of V TG at V BG =−10 V, showing the chirality-assisted decoupling regime. The interface separates BLG-like electron and hole-doped regions (inset), and the measured conductance shows only small-amplitude fluctuations (see also Supplementary Fig. S4 ). ( d ) Calculated transmission probability at a single pn interface for the electrostatic conditions in ( c ). In this regime, transmission probability is dominated by BLG–BLG anti-Klein tunnelling: the pseudospin mismatch between k || =0 holes in the GL and k || =0 electrons in the LGR suppresses transmission through the RBS [28] , resulting in a dip in the normal transmission probability and, ultimately, the suppression of the giant oscillations. Full size image Transmission amplitudes and the conductance oscillations Oscillatory conductance in an electronic Fabry-Pérot etalon arises from quasiparticle trajectories that have comparable reflection and transmission amplitudes: too transmissive, and the particles are never trapped under the barrier, too reflective and they never enter from the lead. At the same time, some selectivity in the angular transmission is necessary to avoid destructive phase averaging, which arises from the random injection angle of quasiparticles incident from the diffusive GLs. Phase coherent transport across the LGR is thus strongly influenced by the transmission properties of the pn junctions defining the LGR, which determine the subset of available states through which ballistic transport can occur. In a ballistic pn junction, the transmission amplitude, T , receives both a semiclassical and a fully quantum contribution [20] , [22] , [23] : | T |~| T SC |·| T Q |. The semiclassical contribution, | T SC |, arises from the conservation of energy and the momentum parallel to the symmetric barrier, k || . In a pn junction, the restricted Fermi surface at the centre of the junction leads to purely evanescent transmission over the region where the local Fermi momentum [22] , | k F ( x )|<| k || |, results in preferential transmission of near normally incident quasiparticles with | k || |~0. When electron wavefunctions do not have a pseudospin structure, | T SC | generally suffices to describe barrier transmission. In chiral electron systems, however, transmission also depends on the existence of a finite matrix element between incident and scattering states [22] , [24] . Chiral particles have a fixed relationship between band index, momentum and pseudospin, the relative phase on the different carbon sublattices, leading to nontrivial contributions to T Q . In MLG, for example, T Q gives rise to the perfect transmission of quasiparticles normally incident on a pn junction (Klein tunnelling), whereas in BLG, the opposite occurs (anti-Klein tunnelling), with transmission forbidden at normal incidence [24] , [25] . Uniquely, TLG allows us to experimentally tune the chiral structure of the wavefunctions through the electric-field tunability of the band structure, allowing us to characterize the role of pseudospin in quasiparticle scattering. Quantitative modelling of the giant oscillations, and their rapid disappearance as a function of both gate voltages and magnetic field, follows from the phase coherent Landauer formula [20] for the conductance, where θ is the phase accumulated by carriers as they traverse the LGR [20] , [26] . We find that equation 1 accounts very well for the conductance oscillation period and relative amplitude with respect to variation of the carrier density and magnetic field (see Fig. 3a–c , and discussion below). The only inputs needed are the electrostatic profile in the device (calculated by finite element analysis) and the TLG band structure [13] , [27] (see Supplementary Discussion), both obtained independently. 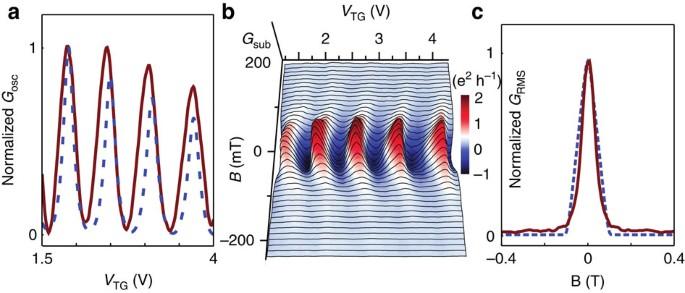Figure 3: Classical confinement of the RBS. (a) Comparison between measured (solid-red) and simulated (dashed-blue) normalized conductance oscillations (Gosc) in the RBS channel at zero magnetic field (B). (b) Magnetic field dependence of the giant oscillations at back-gate voltage (VBG) 1.6 V. The oscillations decay rapidly with magnetic field, indicating a shift to transport channels that do not include the RBS. The average conductance,, over the displayed gate voltage range has been subtracted from the conductance,G(B), at each constantBtrace to remove the strong magnetic field dependence of the GL resistance:. (c) Comparison between normalized conductance amplitude of the measured (solid-red) and simulated (dashed-blue) oscillations as a function of magnetic field. The simulations reproduce the observed rapid decay in oscillation amplitude due to classical confinement, in which collapse of the giant oscillations occurs as, whereBCis the critical magnetic field,is the Fermi momentum in the GL,Lis the size of the LGR,is Plank’s constant divided by 2π andeis the elementary charge. Figure 3: Classical confinement of the RBS. ( a ) Comparison between measured (solid-red) and simulated (dashed-blue) normalized conductance oscillations ( G osc ) in the RBS channel at zero magnetic field ( B ). ( b ) Magnetic field dependence of the giant oscillations at back-gate voltage ( V BG ) 1.6 V. The oscillations decay rapidly with magnetic field, indicating a shift to transport channels that do not include the RBS. The average conductance, , over the displayed gate voltage range has been subtracted from the conductance, G ( B ), at each constant B trace to remove the strong magnetic field dependence of the GL resistance: . ( c ) Comparison between normalized conductance amplitude of the measured (solid-red) and simulated (dashed-blue) oscillations as a function of magnetic field. The simulations reproduce the observed rapid decay in oscillation amplitude due to classical confinement, in which collapse of the giant oscillations occurs as , where B C is the critical magnetic field, is the Fermi momentum in the GL, L is the size of the LGR, is Plank’s constant divided by 2π and e is the elementary charge. Full size image Analysis of equation 1 shows that two factors, absent in other graphene-based interferometers, conspire to enhance the amplitude of the giant oscillations. First, the sum in (equation 1) runs over momenta corresponding to propagating states in both the GLs and LGR, . In the giant oscillation regime, the Fermi surface in the GLs is small in comparison with that in the LGR, leading to an effective collimation of the trajectories within the barrier. Second, the interflavour nature of the MLG–BLG interface suppresses strong contributions to T Q , which is approximately angle independent, with transmissivity of ~50% ( Fig. 2b ). The Fermi surface mismatch thus serves to preferentially inject carriers into the near-normal RBS in the junction, whereas the weak angular dependence and ~1/2 value of the pseudospin matrix element ensures that transmission is in the optimal range, leading to the large observed oscillation amplitudes. Quantum confinement of the resonant states The giant oscillations are sensitive to small changes in the density in the GLs (see Fig. 1c ). Figures 2a and c show fixed − V BG conductance traces in and out of the giant oscillation regime. Electrostatics simulations show that the sudden disappearance of the oscillations at high GL density coincides with a transition in the pseudospin structure of the GL wavefunctions: the oscillations are quickly suppressed once the BLG-like bands start to become occupied in the GLs (see insets in Fig. 2a and c ). The nature of this suppression can be traced to the effect of BLG anti-Klein tunneling [21] , [23] , [24] on T Q . Although for the MLG–BLG interface, carriers are injected predominantly into the low k || RBS, the BLG–BLG interface features a chiral mismatch between low k || states on opposite sides of the barrier. Fig. 2b–d show numerical simulations of the pn junction transmission amplitudes for values of the GL density corresponding to the traces in Fig. 2a–c . The qualitative change in the total pn junction transmission is visible as a shift from high transmission to near-complete reflection at normal incidence: in the BLG–BLG regime, the RBS are effectively decoupled due to chiral mismatch to the leads. Although it is the tunable carrier chirality in ABA TLG that makes this effect observable in the current experiment, ‘anti-Klein’ tunnelling is a generic feature of chiral carriers with 2π Berry phase, such as those in BLG. Classical confinement of the resonant states The decoupling of the RBS can also be achieved by a classical mechanism through the application of an out-of-plane magnetic field, B . Fig. 3b shows the B dependence of the giant oscillations: they disappear rapidly with B , and are completely suppressed by B ~100 mT. This is in stark contrast to the Fabry-Pérot oscillations observed in MLG [16] , [20] , and the smaller Fabry-Pérot oscillations faintly visible in Fig. 1d , which survive up to high B (see Supplementary Fig. S4 ). The disappearance of the giant oscillations with B can be tied to a classical version of the confinement of the RBS, facilitated in TLG by the widely tunable Fermi surface area. The magnetic field exerts a Lorentz force on particles traversing the LGR (see Fig. 4 ). During the resulting cyclotron motion, k || is no longer conserved as the carriers cross the LGR, and change with coordinate [28] : , where x 1 and x 2 denote the positions of the two pn junctions and L = x 2 − x 1 . However, with the exception of small corrections [29] , k || is still conserved in the tunnelling process at a single pn junction. Classical decoupling occurs when this condition can no longer be satisfied (see Fig. 4c ). Because the giant oscillations are observed in a regime of extreme Fermi surface mismatch ( ), only a small magnetic field is necessary to make simultaneous momentum and energy-momentum conservation impossible at the second interface, . Fig. 4 shows the three distinct magnetic field regimes schematically. For small values of B , the field simply introduces a difference in the incident angle of a quasiparticle trajectory on the two junctions for most values of k || (see Fig. 4b ). However, above a critical magnetic field, , the field imparts such a large transverse momentum to the carriers in the RBS that they can no longer escape to the GLs, and effectively decouple from transport (see Fig. 4c ). As in the case of chirality-assisted confinement described above, the resulting decoupling of the RBS from the lead states drives transport to diffusive channels, in which impurity scattering in the LGR provides the momentum relaxation required for quasiparticle escape. 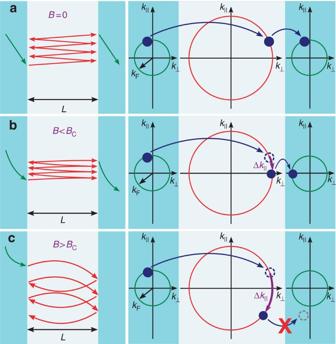Figure 4: Schematic illustration of the classical magneto-decoupling of the RBS. (a) At zero magnetic field (B), carriers are injected from the GL into low parallel momentum (k||) states in the LGR, resulting in transport through the RBS and giant oscillations in the resistance. (b) As the magnetic field increases, quasiparticles gain, as they cross the LGR;Lis the size of the LGR,is Plank’s constant divided by 2π andeis the elementary charge. Although trajectories for whichare excluded from ballistic transport, some ballistic transport is still possibleviathe RBS;is the Fermi momentum in the GLs. (c) For magnetic field larger than the critical magnetic field,, ballistic transportviathe RBS is no longer possible. Charge transport proceeds by momentum nonconserving channels that do not involve the RBS, likely mediated by impurity scattering within the LGR, and the giant oscillations disappear. Figure 4: Schematic illustration of the classical magneto-decoupling of the RBS. ( a ) At zero magnetic field ( B ), carriers are injected from the GL into low parallel momentum ( k || ) states in the LGR, resulting in transport through the RBS and giant oscillations in the resistance. ( b ) As the magnetic field increases, quasiparticles gain , as they cross the LGR; L is the size of the LGR, is Plank’s constant divided by 2π and e is the elementary charge. Although trajectories for which are excluded from ballistic transport, some ballistic transport is still possible via the RBS; is the Fermi momentum in the GLs. ( c ) For magnetic field larger than the critical magnetic field, , ballistic transport via the RBS is no longer possible. Charge transport proceeds by momentum nonconserving channels that do not involve the RBS, likely mediated by impurity scattering within the LGR, and the giant oscillations disappear. Full size image ABA TLG constitutes a high mobility and highly tunable electronic system: carrier density, Fermi surface area, energy-momentum dispersion, quasiparticle chirality and pseudospin can all be tuned electrostatically over large ranges. In this article, we have used this tunability to realize a novel Fabry-Pérot interferometer device, where we explore both quantum confinement of chiral carriers and the limits of semiclassical magnetoconfinement in nanostructures. These phenomena and the unique versatility of TLG hold promise for the realization of devices with novel functionality based on pseudospintronics. Preparing flat encapsulated devices Encapsulated ABA TLG devices are fabricated by exfoliating hBN and graphene flakes on polymer-coated substrates and by transferring them using the flip-chip bonding technique described by Taychatanapat et al. [13] The device shown in Fig. 1a is fabricated by exfoliating a 30-nm thick hBN on top of a 285-nm thick SiO 2 . The atomic flatness of the hBN surface is verified by atomic force microscopy (AFM). A TLG graphene flake is transferred atop of the hBN by using the flip-chip bonding method. The TLG height is verified by AFM ( h =1.1±0.1 nm), and its ABA staking order is confirmed both by Raman spectroscopy and later by quantum Hall measurements, where the characteristic intersecting fans of MLG/BLG Landau levels are observed [13] . Before the encapsulating procedure, we deposit electrical contacts using electron beam lithography and thermal evaporation of Cr/Au contacts at low pressure ( P =10 −7 Torr). The sample is annealed in forming gas (H 2 :Ar—300:700 sccm) at 573 K to remove polymer residues, and then the flat, clean and bubble-free TLG is encapsulated by a (12.5±0.5)-nm thick hBN; also transferred by flip-chip bonding. It is worth noting that the flatness of the hBN and the cleanness of the graphene are essential to avoid carrier inhomogeneity and obtain high-mobility samples. Indeed the presence of bubbles on the TLG is strongly undesired because they can induce strain and create distortions in the ABA band structure [30] . Top-gate fabrication It is common to observe bubbles in the final transferred hBN layer. These can cause inhomogeneity in the capacitive coupling to the top gate. Care is taken to map out the bubbles using AFM before the final design of the top-gate eletrode, so that the resulting 60-nm wide top-gate electrode lies atop an hBN-TLG-hBN stack of uniform thickness. How to cite this article: Campos, L.C., et al. Quantum and classical confinement of resonant states in a trilayer graphene Fabry-Pérot interferometer. Nat. Commun. 3:1239 doi: 10.1038/ncomms2243 (2012).